Complete gate control of supercurrent in graphenep–njunctions In a conventional Josephson junction of graphene, the supercurrent is not turned off even at the charge neutrality point, impeding further development of superconducting quantum information devices based on graphene. Here we fabricate bipolar Josephson junctions of graphene, in which a p – n potential barrier is formed in graphene with two closely spaced superconducting contacts, and realize supercurrent ON/OFF states using electrostatic gating only. The bipolar Josephson junctions of graphene also show fully gate-driven macroscopic quantum tunnelling behaviour of Josephson phase particles in a potential well, where the confinement energy is gate tuneable. We suggest that the supercurrent OFF state is mainly caused by a supercurrent dephasing mechanism due to a random pseudomagnetic field generated by ripples in graphene, in sharp contrast to other nanohybrid Josephson junctions. Our study may pave the way for the development of new gate-tuneable superconducting quantum information devices. A graphene layer [1] , [2] , a one-atom-thick planar sheet of carbon atoms, attached to two closely spaced superconducting electrodes forms a Josephson junction (JJ) [3] , in which the supercurrent flows through graphene via coherent electron–hole Andreev pairs [4] . For earlier discussions on the proximity-induced superconductivity, please refer to ref. 5 and references therein. As a JJ can be described in terms of motion of superconducting phase particles in a potential well [6] , macroscopic quantum tunnelling (MQT) [7] and energy level quantization [8] , which have already been observed in a JJ of graphene (JJG) [9] , provide essential requisites for superconducting quantum bits [6] in graphene. In a JJG, however, complete switching off of the junction supercurrent by the gate voltages has not yet been achieved. This incomplete gate control of the supercurrent in a JJG [4] , [9] , [10] , [11] poses an obstacle in the way of quantum-state engineering. From a fundamental viewpoint, a JJG is rich in physics, providing the opportunity to study the Josephson effect combined with relativistic Dirac nature, as low-energy quasiparticles in graphene are described by massless Dirac fermions [12] . A recent theoretical work [13] showed that a finite supercurrent flows through a JJG in the ballistic regime in the absence of an external magnetic field; this occurs even when the Fermi energy is tuned to the charge neutrality point (CNP; that is, the centre of a Dirac cone) with nominal zero carrier density. In this case, the product of the Josephson critical current I c and the normal-state resistance R n is within an order of Δ / e near the CNP, satisfying the conventional Ambegaokar–Baratoff relation [14] . It has also been shown [15] that specular Andreev reflections occur at the graphene-superconductor interface near the CNP, due to the Dirac-cone energy band structure. However, the effects of intrinsic scattering sources in graphene on the supercurrent of a JJG have not been studied in detail [16] . The role of the valley degrees of freedom on scattering of supercurrent flow in graphene has not been explored. In addition, it would be interesting to investigate a JJG with an electrostatic potential barrier in its normal region; the presence of a potential step is known to induce the negative refraction and Klein tunnelling of Dirac fermions [17] , [18] , with the latter being analogous to the behaviour of relativistic particles. Understanding such scattering effects would be highly useful for graphene-based supercurrent device development. Here we report complete switching off of the supercurrent in a p–n junction of graphene by dual operation of the top and bottom gates. This supercurrent OFF state does not necessarily require an infinite junction resistance by reduced carrier density in the normal state, which is in marked contrast to other hybrid JJs of nanomaterials [19] , [20] , [21] , [22] . Gate-driven crossover of the escape processes of superconducting phase particles, from MQT to the classical regime, is also demonstrated as a novel route for manipulating the macroscopic quantum states. We suggest that the spatially random pseudomagnetic field generated by the ripples (spatially non-uniform strain) in graphene is mainly responsible for the observed supercurrent OFF state. The ripples act as intravalley scattering sources. The random pseudomagnetic field can cause dephasing of coherent Andreev electron–hole pairs in the normal region of the junction, possibly leading to full suppression of the junction supercurrent near the CNP and in the bipolar junction region of the gate voltages, where scattering by ripples becomes most significant. The evidence of ripples in our junction was supported by weak antilocalization (WAL) analysis, which showed that the scattering rate by ripples was substantially enhanced near the CNP. Our study provides a key step towards developing superconducting quantum information devices [23] , [24] based on graphene technology [12] . Gate-controlled complete suppression of I c in a bipolar JJG A schematic view of the bipolar JJG is shown in Fig. 1a , where the JJG is sandwiched between the local top-gate ( V tg ) and global back-gate ( V bg ) electrodes (see Methods for device fabrication). In the superconducting state at the base temperature ( T ~50 mK), the current−voltage ( I – V ) characteristics in Fig. 1b , with V tg =0 V, clearly show supercurrent branches; here the critical (or switching) current ( I c ) reaches 500 nA in the highly p -doped region. Complete I c suppression is obtained at the CNP, corresponding to V bg =12.5 V. Varying V tg and V bg in a stepwise manner, we obtain the colour plot of I c in Fig. 1c , which resembles a quadrant map of the normal-state conductance G (= R n −1 ) showing four distinct regions of junction states: p–p ′, p–n , n–p and n–n ′. These states depend on the respective carrier types under the influence of V bg and V tg (see Supplementary Figs S1 and S2 ). It should be emphasized that I c vanishes completely at the CNP and inner parts of the bipolar region as well. The slice plots in Fig. 1d show that the supercurrent OFF state is obtained even with relatively low values of R n (~0.3 kΩ); this corresponds to a sheet conductance of G sq ~13 e 2 / h , where e is the elementary charge and h is Planck’s constant. 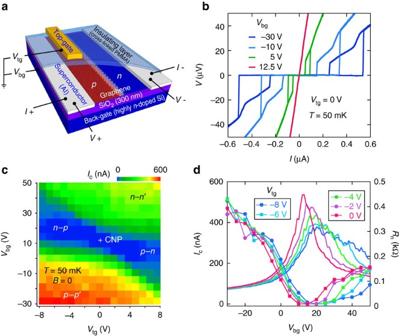Figure 1:Gate-controlled complete suppression of supercurrent inJA. (a) Schematic configuration of the JJGp–nbarrier (JA) established by the dual-gate operation ofVbgandVtg. (b)Vbgdependence of the junction critical current (Ic) and retrapping current (Ir) at the base temperature andB=0, withVtgfixed at 0 V. Highly doped states exhibit a clearIcwith large hysteresis. (c) Colour-coded plot ofIctaken atB=0. The quadrant map ofIcwas obtained from theI–Vcurves by varyingVbgandVtgby steps of 5 and 1 V, respectively. The overall CNP forms atVbg=12.6 V andVtg=0 V. (d)Vbgdependence ofIc(symbol) and the normal-state resistanceRn(line) forVtg=0, −2, −4, −6 and −8 V. Figure 1: Gate-controlled complete suppression of supercurrent in J A . ( a ) Schematic configuration of the JJG p–n barrier ( J A ) established by the dual-gate operation of V bg and V tg . ( b ) V bg dependence of the junction critical current ( I c ) and retrapping current ( I r ) at the base temperature and B =0, with V tg fixed at 0 V. Highly doped states exhibit a clear I c with large hysteresis. ( c ) Colour-coded plot of I c taken at B =0. The quadrant map of I c was obtained from the I–V curves by varying V bg and V tg by steps of 5 and 1 V, respectively. The overall CNP forms at V bg =12.6 V and V tg =0 V. ( d ) V bg dependence of I c (symbol) and the normal-state resistance R n (line) for V tg =0, −2, −4, −6 and −8 V. Full size image When a microwave field with frequency f mw is applied, the I–V curve exhibits quantized voltage plateaus, or Shapiro steps (SSs) [14] , occurring at V n = nhf mw /(2 e ) with integer n , due to phase locking between the JJG and microwave ( Supplementary Fig. S3 ). Typical standard Josephson effects, including SSs and periodic modulation of the I c with a perpendicular magnetic field (that is, Fraunhofer pattern [14] ), are obtained in the overdoped unipolar region ( Supplementary Fig. S3 ). When V bg is varied from the overdoped n–n ′ region to the CNP with V tg =0 V, progressive evolution of the dI / dV peaks, equivalent to the SSs, is evident as shown in Fig. 2a for a fixed microwave power ( P ). 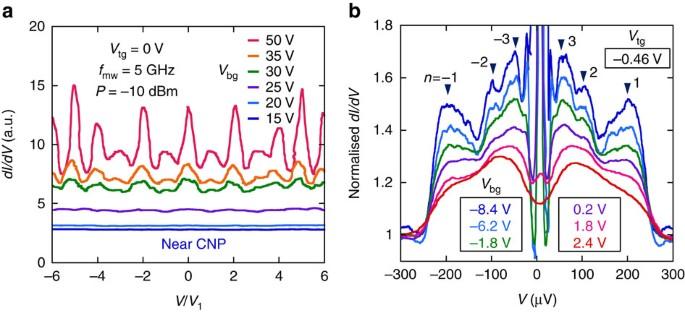Figure 2: Suppression of SSs and MARs near CNP of graphene. (a) Progressive evolution of the differential conductance of the junctionJA, under the irradiation of a microwave of frequencyfmw, with varyingVbgforVtg=0 V, with peaks occurring at the bias voltageVfor integral multiples ofV1(=hfmw/2e=10.3 μV). ThedI/dVpeaks, equivalent to SSs, are completely suppressed as the CNP (Vbg=12.5 V forVtg=0 V) is approached. (b) Progressive change ofdI/dVversusVcurve of the junctionJBas the CNP is approached. ThedI/dVvalue is normalized by the normal-state resistanceRnfor eachVbg. The conductance enhancement at the subharmonic voltages, reflecting the MARs, is suppressed and the supercurrent at zero-bias voltage converts into a dip ofdI/dVnear the CNP. Figure 2a clearly shows that the SSs are absent near the CNP, in contrast to the previous report of significantly reduced but still finite SSs in the plain JJG [11] . The vanishing SSs are attributed to complete I c suppression at the CNP in this experiment. The SSs also vanish in the bipolar n–p and p–n region ( Supplementary Fig. S4 ). Figure 2: Suppression of SSs and MARs near CNP of graphene. ( a ) Progressive evolution of the differential conductance of the junction J A , under the irradiation of a microwave of frequency f mw , with varying V bg for V tg =0 V, with peaks occurring at the bias voltage V for integral multiples of V 1 (= hf mw /2 e =10.3 μV). The dI / dV peaks, equivalent to SSs, are completely suppressed as the CNP ( V bg =12.5 V for V tg =0 V) is approached. ( b ) Progressive change of dI / dV versus V curve of the junction J B as the CNP is approached. The dI / dV value is normalized by the normal-state resistance R n for each V bg . The conductance enhancement at the subharmonic voltages, reflecting the MARs, is suppressed and the supercurrent at zero-bias voltage converts into a dip of dI / dV near the CNP. Full size image Additional experimental evidence for complete I c suppression is shown in Fig. 2b , displaying the dI / dV versus V curve with respect to V bg . With V bg =−8.4 V in the p–p ′ region, we observe multiple dI / dV peaks occurring at V =2 Δ / ne , where 2 Δ =210 μeV is the superconducting energy gap of Al. These subgap conductance peaks are due to the multiple Andreev reflection (MAR) effect [4] , [10] , [25] , where the electron-like quasiparticle in a normal metal (N), incident to the superconductor (S), is retro-reflected as a phase-conjugated hole-like quasiparticle at the N–S interface, leaving Cooper pairs in S and vice versa. When V bg approaches the CNP ( V bg =2.4 V for device J B ), the infinitely high dI / dV peak, corresponding to a finite supercurrent, converts into a zero-bias dI / dV dip; this is consistent with the observations of the supercurrent OFF state formed near the CNP. We note that the MAR is also suppressed, resulting in a substantial decrease of the dI / dV peak heights near the CNP, in contrast with a previous report [10] of MAR peaks that were insensitive to V bg in a plain JJG. Similar gradual suppression of MAR peaks is seen as V tg approaches the bipolar junction region for fixed V bg =5 V ( Supplementary Fig. S4e ). Our observation suggests that the phase-coherent transport of the Andreev-reflected quasiparticle pairs is hindered at the I c suppression region. Theoretically, it is expected [13] , [26] that a JJG can carry a non-zero supercurrent even at the CNP, where the charge density is tuned to zero. In this case, the I c R n product is nearly constant as ~2 Δ / e with V bg in a ballistic short junction [13] , which is in essence the Ambegaokar–Baratoff relation [14] ; in a diffusive long junction, it is given by αE Th / e (refs 11 , 27 ), where E Th is the Thouless energy and α is a coefficient depending on E Th / Δ . Previous experiments [4] , [9] , [10] , [11] of JJG in a diffusive junction regime have shown that the I c R n product at the CNP is almost half the maximum value obtained in the overdoped region. As our bipolar JJG exhibits the maximum I c R n =40 μV in the overdoped region, the minimum I c is expected to be ~44 nA from R n =450 Ω at the CNP. This discrepancy, between the expected value of I c and the observed completely suppressed value, is not explained by thermal fluctuations [11] . Thermal suppression of I c by 2 nA is estimated for T =50 mK, by comparing the Josephson coupling energy ( E J = ħI c /2 e ; ħ = h /2π) and thermal energy [14] ( k B T ). Environmental noise or low transparency at the junction interface is ruled out by considering a maximum I c ~500 nA in the overdoped region, sufficiently larger than previously reported values [4] , and clear existence of the MAR peaks. A possible mechanism for the supercurrent OFF state is discussed below. Temperature- and gate-dependent current-switching behaviour Complete gate control of the supercurrent in the bipolar JJG would significantly facilitate the gate-tuneable operation of macroscopic quantum states in the JJ, where the confinement energy of superconducting phase particles is determined by E J . As the MQT of the phase particle, a direct evidence of macroscopic quantum state existing in the JJ, is determined by competition between E J and k B T , the gate tuneability of I c in the bipolar JJG would allow the escaping process of the phase particle to be controlled using the gate voltages only. The switching distribution of I c is used to reveal the escaping process in the JJ (see Fig. 3a ). Temperature-dependent I c distributions of the bipolar JJG with fixed V bg and V tg are fitted well to the theoretical models of phase diffusion (PD), thermal activation (TA) and MQT in sequence (see Fig. 3b and Supplementary Fig. S5 ), which are quite similar to the previous observations using the plain homogeneous JJG [9] . Surprisingly, the progressive change of the I c distribution is also obtained with varying V bg for fixed temperature, as shown in Fig. 3c . The theoretical models of PD, TA and MQT fit well the experimental data, revealing that sequential crossover of the escaping processes is tuned by V bg instead of temperature. To the best of our knowledge, this work is the first to demonstrate full control of the phase particle’s escaping process using the gate voltage only. Similar behaviour of the gate-tuned I c distribution curve is also observed with different V tg (see Supplementary Fig. S6 ). This achievement is attributed to the complete gate tuneability of the I c to render a significant variation of the ratio between k B T and E J at a fixed temperature. 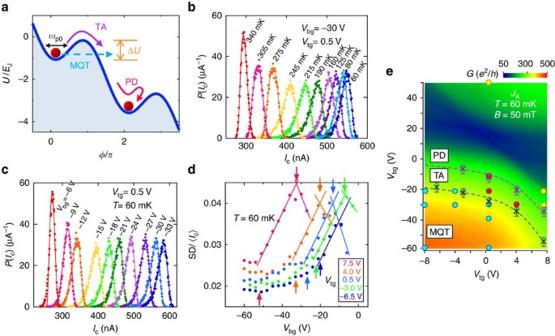Figure 3:T- andVbg-driven current switching of bipolar JJG (JA). (a) Schematic of washboard potentialU(φ) normalized by the Josephson coupling constantEJ(φis the phase difference across the JJ) and dynamics of a phase particle escaping from the local potential minimum (PD, phase diffusion; TA, thermal activation; and MQT, macroscopic quantum tunnelling). (b)Tdependence of the switching current distributionP(Ic) of the JJG,JA, for fixedVbg(=−30 V) andVtg(=0.5 V). The solid lines are the best fits to the PD (T=245~340 mK), TA (T=125~215 mK) and MQT (T=60, 80 mK) model. (c)Vbgdependence of the switching current distribution for fixedVtg(0.5 V) atT=60 mK. The solid lines are the best fits for PD (Vbg=−6~−12 V), TA (Vbg=−15~−24 V) and MQT (Vbg=−27~−33 V) models, respectively. (d) Normalized s.d. versusVbgplot for differentVtgatT=60 mK, extracted from the distributions inFig. 3candSupplementary Fig. S6. Lines are guides for the eye. Upward and downward arrows represent the crossover back-gate voltages between the MQT and TA regions (Vbg,q) and between the TA and PD regions (Vbg,p), respectively, for the given fixed values ofVtg. (e) The quadrant conductance map overlaid with the MQT, TA and PD regions of the switching-current distribution in thep–p' state of graphene ofJA. Cross symbols represent the crossover gate voltages determined fromFig. 3d. Dashed lines are guides for the eye. The filled circular symbols denote the points where theTdependence of the s.d. given inFig. 7. Cyan (red, yellow)-filled circles represent the MQT (TA and PD) regime at the base temperature, which is determined by theTdependence of normalized s.d. Figure 3: T - and V bg -driven current switching of bipolar JJG ( J A ). ( a ) Schematic of washboard potential U ( φ ) normalized by the Josephson coupling constant E J ( φ is the phase difference across the JJ) and dynamics of a phase particle escaping from the local potential minimum (PD, phase diffusion; TA, thermal activation; and MQT, macroscopic quantum tunnelling). ( b ) T dependence of the switching current distribution P ( I c ) of the JJG, J A , for fixed V bg (=−30 V) and V tg (=0.5 V). The solid lines are the best fits to the PD ( T =245~340 mK), TA ( T =125~215 mK) and MQT ( T =60, 80 mK) model. ( c ) V bg dependence of the switching current distribution for fixed V tg (0.5 V) at T =60 mK. The solid lines are the best fits for PD ( V bg =−6~−12 V), TA ( V bg =−15~−24 V) and MQT ( V bg =−27~−33 V) models, respectively. ( d ) Normalized s.d. versus V bg plot for different V tg at T =60 mK, extracted from the distributions in Fig. 3c and Supplementary Fig. S6 . Lines are guides for the eye. Upward and downward arrows represent the crossover back-gate voltages between the MQT and TA regions ( V bg,q ) and between the TA and PD regions ( V bg,p ), respectively, for the given fixed values of V tg . ( e ) The quadrant conductance map overlaid with the MQT, TA and PD regions of the switching-current distribution in the p–p ' state of graphene of J A . Cross symbols represent the crossover gate voltages determined from Fig. 3d . Dashed lines are guides for the eye. The filled circular symbols denote the points where the T dependence of the s.d. given in Fig. 7 . Cyan (red, yellow)-filled circles represent the MQT (TA and PD) regime at the base temperature, which is determined by the T dependence of normalized s.d. Full size image Three distinctive regimes of the switching process can be identified using the standard deviation (s.d.) of the I c distribution normalized by the mean value I c , as shown in Fig. 3d , depending on V bg and V tg . The switching rate in the TA regime, Γ TA ~exp(− I c ), is more sensitive to the I c than that of the MQT where Γ MQT ~exp(− I c 0.5 ). Thus, we can define the crossover gate voltage of V bg,q , between the MQT and TA regions, as the value of V bg at which the slope of the normalized s.d. changes abruptly [9] . A second crossover gate voltage ( V bg,p ) between the TA and PD regions is defined as V bg when the slope changes its sign. An overlay of the I c switching mechanism phase diagram on the quadrant map of G is shown in Fig. 3e , where the crossovers between the switching processes are fully gate driven in contrast to the plain JJG [9] . We note that the phase boundary lines are shifted from the boundary of the quandrant map, forming the contour line of I c for each crossover. This also indicates that the competition between E J and k B T is responsible for the crossovers. Supercurrent suppression mechanism A typical turning-off process of the supercurrent in other nanohybrid JJs [19] , [20] , [21] , [22] utilizes an infinite R n induced by carrier depletion in the nanostructures. I c suppression in the bipolar JJG, however, is not accompanied by a divergent R n , alluding the unusual turning-off mechanism for the supercurrent. This could be caused by selective transmission of carriers in Klein tunnelling [17] , [18] , which hinders the phase-coherent propagation of the Andreev-reflected quasiparticle pairs at the p–n boundary, or by specular-like reflection at the interface between charge puddles [16] . The latter effect by charge puddles changes the dynamical phase of the charge carriers in the normal graphene region; hence, it can give rise to dephasing of the Andreev-reflected quasiparticle pairs. However, the change in the dynamical phase is not expected to be sufficient to cause dephasing in the short junction limit, where the superconducting coherence length, ξ s (=( ħD / Δ ) 1/2 =260 nm), is comparable to the junction spacing, L (300 nm), with a diffusion constant of D =110 cm 2 s −1 in this study. Moreover, the former effect by Klein tunnelling alone is not sufficient to explain complete I c suppression at the CNP (see Supplementary Figs S7 and S8 ). Here we propose a new I c suppression mechanism, based on ripples and other scattering sources of Andreev quasiparticle pairs, which may exist in our JJG. Our mechanism is summarized as follows. An electron and its Andreev-reflected hole acquire a different amount of phase shift in the normal n–p region, due to spatially random pseudomagnetic fields induced by ripples [28] , [29] . The resulting random phase shifts can cause dephasing of the Andreev pairs, and hence a large reduction in the phase-coherent effect of the Josephson current near the CNP, where scattering by ripples becomes significant. Scattering sources such as puddles [30] , specular Andreev reflection [15] and the interface between n -type and p -type regions [17] , [18] further enhance the reduction, possibly leading to full I c suppression. This suppression in I c occurs, because an electron and its Andreev-reflected hole propagate along different paths that become further deviated from each other due to the scattering sources, and acquire ripple-induced random phase shifts with respect to each other. Ripples, spatially non-uniform strains, are intrinsic structures of graphene [31] and affect the electron properties by inducing pseudomagnetic fields [28] , [29] . In contrast to real magnetic fields, the pseudomagnetic fields are opposite in their direction with respect to the other between the K and K ′ valleys. Thus, although these pseudomagnetic fields break the effective time reversal symmetry defined within a single valley, the actual time reversal symmetry remains intact [32] . A ripple typically has a diameter of d~ 10 nm and a height h R ~0.2 nm [33] , [34] , generating a pseudomagnetic flux, Φ, in the region of the ripple, defined by [28] where Φ 0 = h /2 e is the flux quantum and a =0.14 nm is the interatomic distance in graphene. An Andreev quasiparticle propagating through a ripple acquires a phase shift of 2 πΝ Φ due to the pseudomagnetic flux, where Ν Φ =Φ/Φ 0 . Our JJG (whose junction length and width were ~300 and ~2,000 nm, respectively) could accommodate ~6,000 ripples in its normal region. The ripples were assumed to be randomly distributed spatially in the normal n–p region. Hence, the total phase shift acquired by an Andreev quasiparticle, resulting from multiple scattering events by the randomly distributed ripples over the junction length, L , follows a Gaussian distribution, with variance σ 2 given by where v F is the Fermi velocity, ~ v F /(| k F(F′) | d 2 ) is the scattering rate [35] by ripples in the n ( p ) region and k F(F′) is the electron wave vector in the n ( p ) region. Here, L /(| k F | d 2 ) represents the number of ripples in the area of L /| k F |. If the ripple-induced phase shift of an electron propagating through the normal region is uncorrelated with that of its Andreev partner (the Andreev-reflected hole), then the random distribution of the total phase shift results in severe reduction of the Josephson supercurrent. It is described by the current-phase relation (see Supplementary Note 7 for the detailed derivation) where φ is the phase difference between the two superconducting JJG electrodes. We notice that the Josephson current is significantly suppressed near the CNP, because increases dramatically as k F(F′) vanishes near the CNP. In contrast to the Josephson supercurrent, the quasiparticle propagation in the normal state is not hindered by the ripple-induced dephasing effect, retaining a finite R n even at the CNP, which is consistent with our observations. As described above, equation (3) is derived under the condition of uncorrelated ripple-induced phase shifts between Andreev partners (an electron and its Andreev-reflected hole). This condition is satisfied, because the Andreev partners usually propagate along different paths from each other in the normal regions, acquiring phase shifts that are uncorrelated due to the random spatial distribution of the ripples. Although extremely rare, it is possible that Andreev partners have exactly the same paths (for example, the case with zero excitation energy). This case contributes to I c , as the ripple-induced phase shifts of the Andreev partners cancel each other, because the Andreev partners are in different valleys (for example, an electron in the K -valley and a hole in the K ′-valley) and are affected by the pseudomagnetic fields with directions opposite to each other [32] . In this case, other scattering sources such as puddles [30] , specular Andreev reflection [15] and the interface between n and p [17] , [18] further reduce and may fully suppress I c , because they make the Andreev partners propagate along different paths that deviate from each other [36] . Thus, the ripple-induced phase shifts become uncorrelated between Andreev partners. For example, near the CNP, a puddle results in the deviation of the propagating paths between the Andreev partners. In this case, an electron (hole) undergoes negative refraction at the interface between the p -type ( n -type) region and a zero-doping region formed near the puddle, whereas a hole (an electron) shows normal refraction at the same interface. Our calculation results based on equation (3), along with the experimental parameters of this work, are in good agreement with the experimental data, as shown in Fig. 4a . The I c suppression observed in the bipolar JJG was mainly caused by the ripple-induced dephasing effect of the Andreev-reflected quasiparticle pairs. The dephasing effect was highly enhanced at the CNP, as expected in the ripple scattering model, whereas it was negligible in the unipolar junction region ( Fig. 1c ). The dephasing effect will also be significant in the bipolar junction region. In the bipolar junction region, a localized CNP region forms spatially at the p–n interface or over one-half of the JJG, as the Fermi level aligns with either side of the bipolar potential profile to make the p –0 (or n –0) state. 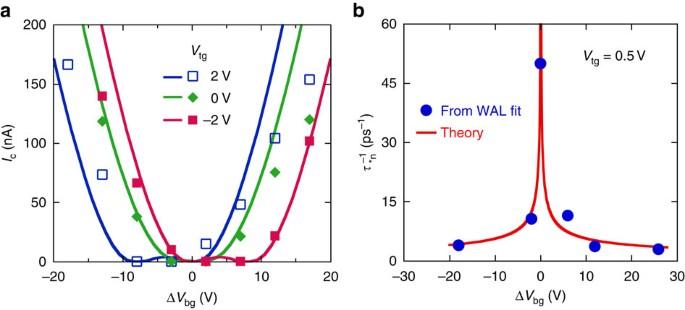Figure 4: Dephasing effect by ripples in graphene. (a) The junction critical currentIc(solid lines) is calculated with varyingVbgwith respect toVCNP(that is, ΔVbg=Vbg−VCNP) at fixed values ofVtgnear the CNP, taking into account the spatially random pseudomagnetic field induced by ripples. The calculation result is in qualitative agreement with the experimental observation fromJA(symbols). (b) Comparison of the scattering rateτ*n−1by ripples (filled circles) as a function of ΔVbg(obtained from a weak-(anti)localization fit forJAatVtg=0.5 V; seeSupplementary Fig. S9) and the theoretical prediction ofτ*n−1~vF/(kFd2) (solid line). Figure 4: Dephasing effect by ripples in graphene. ( a ) The junction critical current I c (solid lines) is calculated with varying V bg with respect to V CNP (that is, Δ V bg = V bg − V CNP ) at fixed values of V tg near the CNP, taking into account the spatially random pseudomagnetic field induced by ripples. The calculation result is in qualitative agreement with the experimental observation from J A (symbols). ( b ) Comparison of the scattering rate τ *n −1 by ripples (filled circles) as a function of Δ V bg (obtained from a weak-(anti)localization fit for J A at V tg =0.5 V; see Supplementary Fig. S9 ) and the theoretical prediction of τ *n −1 ~ v F /( k F d 2 ) (solid line). Full size image WAL analysis To find the evidence of ripples in our JJG, we measured the magnetoconductance of the normal state of the JJG and analysed the WAL effects. As the pseudomagnetic field of the ripples breaks the effective time reversal symmetry within a single valley [37] , the WAL effect [38] in graphene can be suppressed by the intravalley scattering due to ripples. It is known that other intravalley scattering sources, such as puddles, may not be detected by WAL analysis, because they do not cause WAL suppression; in addition, the trigonal warping effect [38] is typically very small (scattering rate ≤0.03 ps −1 ) near the CNP. Therefore, the suppression of WAL at the CNP can be interpreted as an evidence of ripples. The measured magnetoconductance of the normal state of our JJG exhibited the suppression of WAL near the CNP. Magnetoconductance data for a top-gate voltage of V tg =0.5 V and temperature of 4.8 K are plotted in Supplementary Fig. S9 . By analysing the data based on the WAL fit [38] for different V bg , we obtained scattering rates for the normal state, which are summarized in Supplementary Table S1 ; the details of the analysis are given in the Methods section. The intravalley scattering rate in the n ( p ) region, , plotted in Fig. 4b , is well described by Here we use the empirical relation [1] for the n region and for the p region. This behaviour agrees with the theoretical expectation [35] of a scattering rate of ~ v F /(| k F(F′) | d 2 ) by ripples. The fitting result of the lateral size of a ripple ( d =35 nm) is within experimentally reasonable values [33] , [34] (on the order of d =10 nm). These results provide an evidence of the presence of ripples in our JJG. We emphasize that we used the same form of in our mechanism of I c suppression (see equations (2) and (3)), which shows the consistency of our analysis of WAL suppression and I c suppression. In addition, the fitting shows that the intervalley scattering rate (by defects and edges) is two orders smaller than the intravalley scattering rate near the CNP. Moreover, it shows that the intervalley scattering rate does not increase as the system approaches the CNP, which is not consistent with the fact that I c is strongly suppressed near the CNP. Therefore, the WAL data exclude other possible I c suppression mechanisms by intervalley scattering. We emphasize that the Ambegaokar–Baratoff relation holds in graphene, when both the actual time reversal symmetry and the effective time reversal symmetry are preserved. Our findings show that, contrary to disorders in conventional JJs, ripples in graphene can give rise to I c suppression, even in the presence of actual time reversal symmetry, because they break the effective time reversal symmetry (for the role of the symmetries, see Supplementary Note 7 ). Recent theoretical work on JJGs [39] has shown that the pseudomagnetic field, induced by strain, strongly affects Andreev-bound states; in this case, however, the critical current was not fully suppressed, because the pseudomagnetic field was not spatially random. In contrast, the excess resistivity due to ripple scattering in the normal state is given by δρ =( h /4 e 2 )( z 4 / R 2 a 2 ), where z ( R ) is the characteristic height (radius) of the ripple and a =0.14 nm is the interatomic spacing in graphene [40] . Using typical values of R ~5 nm and z ~0.2 nm [33] , [41] , we obtained δρ ~8.3 × 10 −4 h / e 2 , which is much smaller than the maximum sheet resistance of R sheet ~0.13 h / e 2 at the CNP in this experiment. Thus, the influence of ripple scattering on R n is minimal. The origin of the ripples in our JJG is not certain, but presumed to be due to the difference in thermal expansion between the graphene layer and the poly (methyl methacrylate) (PMMA) layer [42] , overlaid for the top-gate insulation, as inferred from the control experiments. We compared two conventional JJGs, with and without a PMMA layer covering the graphene (see Supplementary Fig. S10 ). 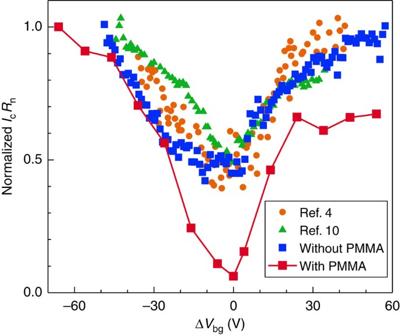Figure 5: Control experiments with homogeneous JJGs. Back-gate voltage dependence of normalizedIcRnproduct (ΔVbg=Vbg−VCNP). The control experimental results from the homogeneous JJG without a PMMA overlayer (blue-filled squares) were very similar to earlier reports from ref.4(circles) and ref.10(triangles), whereas the homogeneous JJG with a PMMA overlayer (Supplementary Fig. S10b, red-filled squares) exhibited substantial suppression ofIcRnat the CNP. Figure 5 displays the V bg dependence of the I c R n product, which is normalized by the maximum value in the overdoped region. The JJG without a PMMA layer clearly exhibited the I c R n product at the CNP, at almost one-half the maximum value in the overdoped region; this tendency has been observed and described in previous reports [4] , [10] , [11] . In contrast, the I c R n product was severely suppressed at the CNP for the JJG with a PMMA layer. This result, consistent with our experimental and theoretical results for the p–n junction, can be explained by ripple-induced I c suppression, with increased ripple density in graphene under the PMMA overlayer. As ripples suppress the supercurrent, but do not significantly affect R n , the conventional version of the Ambegaokar–Baratoff relation does not hold near the CNP in JJGs with ripples, as shown in Fig. 5 . Figure 5: Control experiments with homogeneous JJGs. Back-gate voltage dependence of normalized I c R n product (Δ V bg = V bg − V CNP ). The control experimental results from the homogeneous JJG without a PMMA overlayer (blue-filled squares) were very similar to earlier reports from ref. 4 (circles) and ref. 10 (triangles), whereas the homogeneous JJG with a PMMA overlayer ( Supplementary Fig. S10b , red-filled squares) exhibited substantial suppression of I c R n at the CNP. Full size image In this study, a bipolar JJG realized the complete supercurrent ON/OFF states for the first time as a genuine graphene supercurrent device. Complete control over the I c is attributed to the pseudomagnetic field-induced dephasing of the electron–hole phase-coherent Andreev processes in rippled graphene; this provides a unique route for turning off the supercurrent in JJGs, without sacrificing the junction quality in the supercurrent ON state, nor demanding infinite R n like other nanohybrid supercurrent transistors [19] , [20] , [21] . Completely tuneable hybrid superconductor graphene devices can be used for developing novel superconducting quantum information devices [23] , such as the Cooper-pair beam splitter [24] , [43] for quantum entanglement. Device fabrication The JJGs [3] , [4] used in this study were fabricated using simple mechanical exfoliation [1] , [2] from graphite flakes (NGS Naturgraphit GmbH) in combination with electron-beam nanofabrication techniques [9] , [11] , [44] . Graphite flakes were exfoliated onto a degenerately doped Si substrate capped with a 300-nm-thick oxidation layer. Visual inspection under an optical microscope allows the identification of single-layer flakes of graphene by the characteristic colouration that arises from optical thin-film interference [45] . Superconducting Al electrodes were placed on the graphene layer by conventional electron-beam lithography and subsequent electron-beam evaporation of a Ti/Al/Au trilayer (10/90/5 nm) under a base chamber pressure of 5 × 10 −8 Torr. The single-layer character of the graphene was confirmed by subsequent quantized Hall conductance measurements in a high magnetic field up to 15 T. The Ti layer was deposited to improve the contact of Al to the graphene layer, whereas the Au capping layer was added to protect the Al from oxidation. To electrically insulate the top gate from the graphene layer, a thin layer of PMMA (molecular mass 950 K, 2% in anisole) was spin-coated onto the graphene layer at 4,000 r.p.m. for 30 s, followed by baking at 180 °C for 120 s on a hot plate. The PMMA was then cross-linked [46] , [47] by exposing it to a 20 keV electron beam at a dose [48] of 15,000 μC cm −2 . The unexposed PMMA was removed by soaking the entire device in acetone for 15 min (see the yellow-dotted-line boundary of the insulating layer in Fig. 6b ). Additional fabrication processes using electron-beam lithography, metal deposition and lift-off were required to define a local top gate (with thickness of 5/30 nm (Ti/Au) and line width of ~50 nm), which covered part of the graphene region between the two superconducting electrodes of the device (see Fig. 6a,b ). 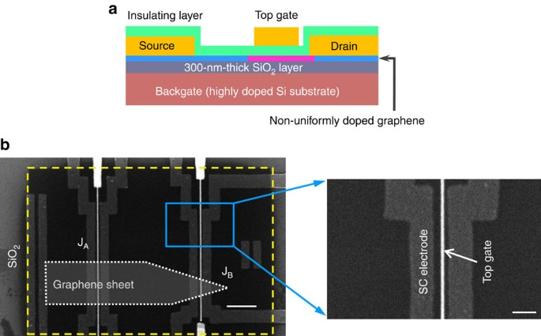Figure 6:Configuration of JJG with ap–nbarrier. (a) Schematic diagram of the side view of the device configuration used in this study. (b) Scanning electron microscopy (SEM) picture of the JJG (devicesJAandJB) with a graphenep–nbarrier (scale bars, 2 μm (left) 0.5 μm (right)). The bright white electrodes applied the top-gate voltage to the graphene layer. White and yellow-dotted lines represent the boundaries of the graphene and the insulating layer for the top gate, respectively. This measurement configuration was used to obtain the data shown inFig. 1a. Figure 6: Configuration of JJG with a p–n barrier. ( a ) Schematic diagram of the side view of the device configuration used in this study. ( b ) Scanning electron microscopy (SEM) picture of the JJG (devices J A and J B ) with a graphene p–n barrier (scale bars, 2 μm (left) 0.5 μm (right)). The bright white electrodes applied the top-gate voltage to the graphene layer. White and yellow-dotted lines represent the boundaries of the graphene and the insulating layer for the top gate, respectively. This measurement configuration was used to obtain the data shown in Fig. 1a . Full size image Low-noise measurements The radio-frequency noise was reduced by adopting a multi-stage filtering scheme: two-stage RC filters (cut-off frequency ~30 kHz) connected in series with leads of a device and silver-powder filters in a cryogenic environment ( T <1 K) in conjunction with π -filters arranged at room temperature. In addition, a small magnetic field was applied to cancel out any residual magnetic fields in the cryostat, allowing zero-field measurements. Figure 6b shows an scanning electron microscopy image of a representative JJG p–n junction device. For the junctions J A and J B , the spacing L between the superconducting electrodes was ~300 nm, while the width W was ~2.2 μm for J A and ~1 μm for J B . A back-gate voltage V bg was applied between the highly electron-doped Si substrate and a graphene layer. This globally modulated the carrier density in graphene to n= α| V bg |, where α ~7.3 × 10 10 cm −2 V −1 for a 300-nm-thick SiO 2 layer [49] on the surface of the substrate. A top-gate voltage V tg was also applied across the PMMA insulating layer. This locally modulated the carrier density in part of the graphene to n ′ =α ′| V tg | beneath the local surface of the insulating layer, where α ′~7.3 × 10 11 cm –2 V –1 for the 30-nm-thick cross-linked PMMA layer [47] , [48] . The dielectric constant of the insulating layer [47] was about ε PMMA =4.5, which is similar to the dielectric constant of SiO 2 . Measurements were carried out at a base temperature of T =50–60 mK, adopting a two-terminal configuration and the conventional ac lock-in technique. In all of our devices, the contact resistance between the graphene and electrode was <1 Ω, which was sufficiently smaller than the resistance of the graphene layer (on the order of a few hundred Ω). Fitting to critical-current-switching models MQT behaviour in a current-biased JJ has been used to develop the superconducting phase qubit [50] . The MQT behaviour in a plain unipolar JJG has been demonstrated [9] using the stochastic distribution of I c , in which the crossover temperature from the classical TA to the MQT regime can be controlled by the application of V bg , thus allowing modulation of the Josephson coupling energy E J . To measure the I c distribution P ( I c ) in our JJG, a saw-tooth-like bias current was applied to the sample through a standard resistor R =10 kΩ with a ramping rate of dI / dt =69 μA s −1 . At the same time, a high-precision 18-bit data acquisition board (NI-6281) recorded 8,000–12,000 switching events with a current resolution of 0.7 nA at a fixed temperature T , a back-gate voltage V bg and a top-gate voltage V tg . A threshold voltage of V th =3 μV was used to determine I c . P ( I c ) measured with a linearly increasing bias current has a well-known relationship with the escape rate Γ of a phase particle trapped in a washboard potential [51] as P ( I c )=[ Γ ( I c )/( dI / dt )]{1— ∫ 0 I c P ( I ′) dI ′}, where φ is the phase difference across the JJ, and I c0 and E J0 (= ħI c0 /2 e ) are the fluctuation-free switching current and Josephson coupling energy, respectively. Γ has different expressions depending on the escape regimes; MQT, TA and PD regimes. The thermal escape rate has an Arrhenius-like temperature dependence as , where a t =(1+1/4 Q 2 ) 1/2 −1/2 Q is a damping-dependent factor, ω p = ω p0 (1− γ 2 ) 1/4 is a Josephson plasma frequency and Δ U =2 E J0 [(1− γ 2 ) 1/2 − γ cos −1 γ ] is the potential barrier height, with quality factor Q =4 I c / πI r , ω p0 =(2 eI c0 /ħ C ) 1/2 and normalized current γ = I / I c0 . Here C is the junction capacitance, a key parameter related to the hysteresis of the I–V curve. In contrast to a superconductor–insulator–superconductor JJ, a proximity JJ of normal metal [52] , carbon nanotubes [21] , semiconducting nanowires [19] , or graphene [4] has negligibly small geometrical capacitance to allow hysteresis. In this analysis, we adopted the effective capacitance C eff originating from the diffusive nature of carriers in graphene, replacing the relaxation time R N C by the diffusion time of Andreev pairs [52] , ħ/ E Th where E Th =ħ D / L 2 is the Thouless energy ( D = v F l /2 is the diffusion constant in graphene, v F is the Fermi velocity, l is the mean free path and L is the junction length) [52] . Γ TA increases exponentially with temperature, which results in broadening of P ( I c ) with increasing temperature. In contrast to Γ TA , the MQT rate does not depend on the temperature explicitly as [7] . Therefore, below the MQT crossover temperature, , Γ MQT overtakes Γ TA and MQT dominates the escape mechanism, resulting in temperature-independent P ( I c ). However, above the PD crossover temperature , a thermally escaped phase particle can be repeatedly retrapped in the following potential well due to strong dissipation. The escape rate Γ PD in the PD regime is modified from Γ TA by retrapping probability [53] P RT as . P RT is obtained from integration of the retrapping rate [54] , [55] , with the retrapping potential barrier Δ U RT ( I )=( E J0 Q 0 2 /2)[( I — I r0 )/ I c0 ] 2 , where I r0 is the fluctuation-free retrapping current and Q 0 =4 I c0 / πI r0 . P ( I c ) in the TA regime has a left-tailed asymmetric shape. In the PD regime, however, the low- I c -tailed feature of P ( I c ) is reduced by the retrapping of an escaped phase particle, resulting in a sharper and more symmetric P ( I c ). 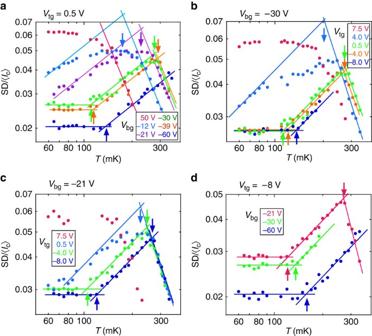Figure 7:Tdependence of s.d. ofP(Ic). Tdependence of the s.d. of the switching-current distributionP(Ic) in the junctionJA, normalized by the junction critical currentIc(a) at fixedVtg=0.5 V, (b) at fixedVbg=−30 V, (c) at fixedVbg=−21 V and (d) at fixedVtg=−8 V. Solid lines are guides for the eyes. Upward and downward arrows represent the crossover temperatures between the MQT and TA regimes (), and those between the TA and PD regimes (), respectively. Figure 7a displays the s.d. of the I c distribution P ( I c ), normalized by ‹ I c › as a function of temperature, while passing through the CNP. In this case, V bg was varied while V tg remained fixed at 0.5 V. Except for the point corresponding to V bg =50 V, all other operation points were in the p–p ′ regime (see Fig. 3e ). The s.d. of the I c distribution was almost constant with respect to temperature in the MQT regime, while increasing (decreasing) with temperature in the TA (PD) regime, similar to the previous observations for a plain unipolar JJG. Here it should be emphasized that the crossover temperatures of (upward arrows) between the MQT and TA regimes, and (downward arrows) between the TA and PD regimes, changed drastically with V bg . When V bg closely approached the CNP, the crossover temperatures tended to shift to much lower temperatures, resulting in the vanishing of down to the base temperature. This feature forms a striking contrast with the MQT behaviour in a plain unipolar JJG, which remains robust even at the CNP. The temperature dependence of the normalized s.d. at the other gate voltages of V bg and V tg in the p–p ′ regime is shown in Fig. 7b,c,d (see circular symbols in Fig. 3e ). The highly sensitive tunability of and with V bg , which is indebted to the fully controllable I c in the JJG, was also observed for different V tg pertaining to the p–n state (not shown). Figure 7: T dependence of s.d. of P ( I c ). T dependence of the s.d. of the switching-current distribution P ( I c ) in the junction J A , normalized by the junction critical current I c ( a ) at fixed V tg =0.5 V, ( b ) at fixed V bg =−30 V, ( c ) at fixed V bg =−21 V and ( d ) at fixed V tg =−8 V. Solid lines are guides for the eyes. Upward and downward arrows represent the crossover temperatures between the MQT and TA regimes ( ), and those between the TA and PD regimes ( ), respectively. Full size image Figure 3e is overlaid with coloured filled-circle symbols that represent the critical current-switching regimes at the base temperature determined by the temperature dependence of normalized s.d. in Fig. 7 . Circular symbols, corresponding to the operation points of the data in Fig. 7 , of a colour belong to a particular switching regime. The switching current regimes, determined by varying temperature at a fixed V bg and V tg in Fig. 7 , are consistent with the boundaries of the different regimes determined by varying V bg at the base temperature in Fig. 3e . WAL analysis We analysed the magnetoconductance measured in our JJG at T =4.8 K, which is above T c , and at V tg =0.5 V. The magnetoconductance of Δ σ = σ ( B )−σ(0) can be described by the series conductance of the two regions, n and p , as where Δ σ n(p) = σ n(p) ( B )− σ n(p) (0) is the magnetoconductance of n ( p ). It is known [38] that the WAL in Δ σ n,p is suppressed, depending on the intravalley scattering rate ( ), intervalley scattering rate ( ) and the dephasing rate ( ) of each region: Here, , ψ is the digamma function, , D n(p) is the diffusion constant determined by the gate voltage applied to n ( p ) and B is the external magnetic field perpendicular to graphene. In equation (5), we introduce a parameter α to compensate for the aspect ratio ( L / W ) associated with the geometry, due to the modification of L by screening of the metallic electrodes and other factors. We chose σ n (0)/( σ n (0)+ σ p (0))≈0.5 as a reasonable value. The scattering rates were obtained by fitting the magnetoconductance data with equation (5) using seven fitting parameters (one for α , three rates for region n and another three for region p , because scattering occurs at different energies for the n and p regions). Note that (i) the number of fitting parameters is effectively four, the minimum number used in most WAL studies, because the rates for the n region are nearly the same as those for the p region in the case of a small V tg ; and (ii) because the digamma function has a sufficiently non-trivial dependence on its argument, the overall factor α is not important in determining the rates in the fitting, because the dependence of equation (5) on B is not governed by α , but by the rates. In the fitting, we used two physically reasonable constraints: (i) that the intervalley scattering rate is smaller than the intravalley scattering rate [56] , and (ii) that all scattering rates are smaller than the momentum relaxation rate [33] , [38] , How to cite this article: Choi, J. -H. et al. Complete gate control of supercurrent in graphene p–n junctions. Nat. Commun. 4:2525 doi: 10.1038/ncomms3525 (2013).